Dido3-dependent HDAC6 targeting controls cilium size Primary cilia are involved in a variety of physiological processes such as sensing of the environment, cell growth and development. Numerous developmental disorders and pathologies arise from defects in these organelles. Multiple proteins that promote formation and disassembly of the primary cilium have been identified, but little is known about the mechanisms that control steady-state cilium size. Here, we show that death inducer obliterator (Dido3)-dependent targeting of histone deacetylase 6 (HDAC6) is a key determinant of cilium size in growth-arrested cells. The amount of either protein negatively correlates with cilium size. Dido3 availability at the centrosome governs ciliary HDAC6 levels, and redistribution of the two proteins controls tubulin acetylation. In turn, basal body localization of Dido3 and HDAC6 depends on the actin network, previously shown to limit cilium size independent of the cell cycle. These results show that not only kinase-dependent activation of a deacetylase but also its subcellular distribution controls substrate selection. Primary cilia are microtubule-based organelles that protrude from the surface of most mammalian cells [1] , [2] . Cilia are involved in a variety of physiological processes; proper timing and maintenance of cilia are considered critical for a variety of cellular processes such as sensing of the environment, cell growth and development [3] , and a direct connection between primary cilia and cancer was proposed recently [1] , [4] . Primary cilia are formed in G0/G1 cells, and ciliogenesis engages the mother centriole for formation of the basal body [5] . As the same structure that supports ciliogenesis is required for formation of a bipolar spindle [6] , cell cycle transitions trigger cilium resorption to allow for reutilization of the centrosome [7] , [8] , [9] . A combination of mitotic kinases promotes cilium disassembly when cells enter S or G2/M phase; especially kinases previously shown to control centrosome function and structure have been assigned this role [10] , [11] , [12] . Whereas some kinases, for example, Nek2 and Mps2, target the basal body during disassembly [12] , [13] , other kinases such as Aurora A and Plk1 act on the microtubule fibres in the cilium stalk [10] , [11] . Aurora A, however, does not seem to phosphorylate cilium-based microtubules by itself. Instead, Aurora A activates histone deacetylase 6 (HDAC6) at the basal body, promoting disassembly of ciliary microtubules through localized tubulin deacetylation. In turn, stimulation of Aurora A depends on a number of upstream activators, among which the HEF-1 scaffold protein [11] , Calmodulin [14] and signalling by the Wnt5a-Plk1 pathway [10] . Together, this combination of mitotic kinases synchronizes resorption of the cilium stalk and reprogramming of the centrosome, thereby promoting formation of a bipolar spindle in the subsequent mitosis. In addition to cell cycle entry and mitosis, cell spreading and contractility allow for cell cycle-independent control of ciliogenesis [15] . In this case, the presence of actin stress fibres in the cell exerts a negative regulatory effect, which can be counteracted by treatment with actin depolymerizing drugs or RNA interference (RNAi) knockdown of actin-anchoring proteins [16] . Although the exact sequence of events linking the actin network to the primary cilium remains unknown, blocking actin polymerization leads to the stabilization of a pericentrosomal compartment in which vesicle trafficking promotes ciliary protein incorporation. In addition, the actin cytoskeleton seems to control a pool of soluble tubulin and thereby availability of building blocks for the cilium stalk [17] . At least one component of the actin network, the Tctex-1 type dynein light chain, synchronizes cilium resorption and S-phase entry [9] , suggesting that also actin redistribution in response to cell spreading might control cilium size. Notwithstanding the recent advances, many details regarding actin-dependent cilium resorption remain undiscovered. Here, we present evidence that several pathways regulating cilium size converge at the level of HDAC6. Tubulin acetylation and deacetylation are key regulators of microtubule stability in mammalian cells [18] , [19] , [20] . HDAC6 controls a wide range of cellular processes in addition to microtubules; subcellular structures for which HDAC6 targets have been identified include the nucleus [21] , autophagosomes [22] and the actin network [23] . Several studies indicate that HDAC6 is actively redistributed to the site of its target proteins [24] , [25] . Local HDAC6 enrichment might thus promote protein deacetylation at the correct subcellular structure. Similarly, HDAC6 accumulation at the primary cilium might contribute to length restriction and resorption of this organelle. We propose a role for Dido3, product of the Death Inducer Obliterator ( Dido ) gene, in actin-dependent HDAC6 delivery to the primary cilium. Dido is expressed in all tissues [26] , and encodes three proteins termed Dido1, -2 and -3 through alternative splicing [27] . Mouse embryonic fibroblasts (MEFs) and other cell types only express the largest isoform, Dido3, indicating that the two smaller splice variants are unnecessary for survival [27] , [28] . Whereas mice tolerate a mutation that eliminates part of the common amino-terminal region, resulting in a truncated protein termed Dido3ΔNT–, deletion of the single exon coding for the Dido3-specific domains is lethal early in development [29] , emphasizing the importance of this isoform. The three isoforms have a common regulatory histone-binding region at their amino terminus, but Dido3 has a specific carboxy-terminal domain involved in subcellular protein targeting [28] , [30] . Dido3 is a centrosome-associated protein, and cells expressing the truncated Dido3ΔNT suffer from centrosome amplification and mitotic spindle defects [28] . The amino-terminal domains deleted in the Dido3ΔNT mutant are involved in retention on the chromatin; Dido3ΔNT ignores these signals, leading to increased availability of the protein in other subcellular compartments [30] , [31] . As Dido3 regulates mitotic microtubules and localizes to the centrosome, it might have a role in regulating microtubule-based organelles in interphase, for example, the primary cilium. We show that the Dido3 protein restricts cilium size in mammalian cells. Whereas an increased amount of Dido3 at the centrosome caused cilium shortening, inhibition of Dido expression by RNAi resulted in elongated cilia. Dido3 controls cilium size through subcellular targeting of HDAC6. The Dido3ΔNT mutation and Dido3 RNAi alter availability of HDAC6 at the basal body and affect tubulin acetylation levels. Furthermore, the subcellular distribution of Dido3 and HDAC6 is dependent on the actin network, because disruption of actin polymerization provokes loss of the two proteins from the basal body. In conclusion, correct subcellular distribution, in addition to activation by kinases, is an important determinant of HDAC6 substrate selection. Dido3-dependent HDAC6 targeting in growth-arrested cells suggests that cell cycle-dependent and -independent pathways regulating cilium size converge at the level of tubulin deacetylation. Dido3 localizes to the basal body in ciliated cells Primary cilia can be formed in a variety of vertebrate cells, including MEFs, by serum starvation-induced growth arrest [32] . Under these conditions, the same subcellular structures that comprise the spindle poles in mitosis—the centrosomes—take on the role of basal body from which the ciliary axoneme projects [4] , [8] . As Dido3, a product of the death inducer-obliterator ( Dido ) gene, accrues at the spindle poles in mitotic cells [28] , this protein might localize to the basal body in MEF that bear a primary cilium. Although Dido encodes three proteins, Dido1, -2, and -3 (ref. 27 ), only Dido3 is expressed in MEF [28] . To determine whether Dido3 localizes to the basal body, primary cilia were induced in MEF and labelled with antibodies against acetylated tubulin (Ac-tub) and Dido3 ( Fig. 1a,b ). As observed before [27] , a large proportion of Dido3 was found in the nucleus. In addition, the antibody detected protein in the cytoplasm and at the base of the primary cilium. Interference with protein production by small interfering RNA similarly suppressed nuclear, cytoplasmic and centrosomal Dido3 signals, confirming antibody specificity. To confirm targeting to the centrosome, V5-tagged Dido3 was expressed in 3T3 cells ( Supplementary Fig. 1 ). V5-tagged Dido3 colocalized with the microtubule-organizing centre in interphase and mitosis, and the Dido3-specific carboxy-terminal domains are sufficient for this localization. These results confirm centrosomal localization of Dido3, and indicate that its carboxy-terminal domain targets the protein to the basal body in ciliated cells. 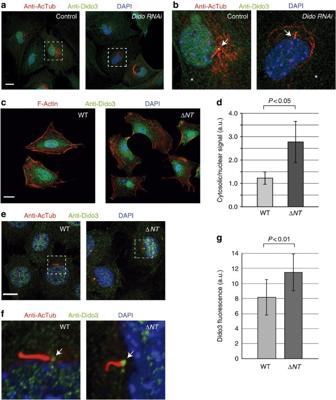Figure 1: Dido3 and Dido3ΔNT show different subcellular distribution. (a) WT mouse embryonic fibroblasts (MEFs) were seeded on coverslips, labelled with anti-Dido3 (green) and Ac-tub antibodies (red), and studied by fluorescence microscopy. DNA was counterstained with 4',6-diamidino-2-phenylindole (DAPI; blue). (b) Magnification of boxed areas ina. (a,b) RNA interference (RNAi) againstDidosimilarly reduced nuclear, cytoplasmic (asterisk) and centrosomal (arrow) signals, confirming antibody specificity. (c) WT or ΔNT MEFs were seeded on coverslips, labelled with anti-Dido3 (green) antibodies, and counterstained for F-actin (red) and DNA (blue). (d) Quantification of nuclear and cytoplasmic signals revealed Dido3ΔNT redistribution to the cytoplasm (one-way analysis of variance (ANOVA)). Error bars indicate standard error of the mean (n=8). (e,f) WT or ΔNT MEFs were seeded on coverslips, labelled with anti-Dido3 (green) and Ac-tub (red) antibodies, and counterstained for DNA (blue). (f) Magnification of boxed areas ine. Note the levels of Dido3 and Dido3ΔNT at the centrosome (arrows). (g) Quantification of Dido3 or Dido3ΔNT levels at the cilium base by one-way ANOVA. Error bars indicate standard error of the mean (n=14). Scale bars, 10 μm. Separate grey scale versions of the micrograph images are supplied inSupplementary Fig. 12. Figure 1: Dido3 and Dido3ΔNT show different subcellular distribution. ( a ) WT mouse embryonic fibroblasts (MEFs) were seeded on coverslips, labelled with anti-Dido3 (green) and Ac-tub antibodies (red), and studied by fluorescence microscopy. DNA was counterstained with 4',6-diamidino-2-phenylindole (DAPI; blue). ( b ) Magnification of boxed areas in a . ( a , b ) RNA interference (RNAi) against Dido similarly reduced nuclear, cytoplasmic (asterisk) and centrosomal (arrow) signals, confirming antibody specificity. ( c ) WT or ΔNT MEFs were seeded on coverslips, labelled with anti-Dido3 (green) antibodies, and counterstained for F-actin (red) and DNA (blue). ( d ) Quantification of nuclear and cytoplasmic signals revealed Dido3ΔNT redistribution to the cytoplasm (one-way analysis of variance (ANOVA)). Error bars indicate standard error of the mean ( n =8). ( e , f ) WT or ΔNT MEFs were seeded on coverslips, labelled with anti-Dido3 (green) and Ac-tub (red) antibodies, and counterstained for DNA (blue). ( f ) Magnification of boxed areas in e . Note the levels of Dido3 and Dido3ΔNT at the centrosome (arrows). ( g ) Quantification of Dido3 or Dido3ΔNT levels at the cilium base by one-way ANOVA. Error bars indicate standard error of the mean ( n =14). Scale bars, 10 μm. Separate grey scale versions of the micrograph images are supplied in Supplementary Fig. 12 . Full size image The amino-terminal domains of Dido3 recognize histone H3, when this protein is trimethylated on lysine 4 (refs 31 , 33 ). In meiosis, histone H3 must be demethylated in order to direct Dido3 to the synaptonemal complex; the amino-terminal segment thus acts as a retention signal that prevents subcellular Dido3 redistribution. Accordingly, a Dido3 mutant that lacks the amino-terminal domains, termed Dido3ΔNT ( Supplementary Fig. 2 ), ignores the trimethylation signal in spermatocytes as detected with an antibody against the carboxy terminus [30] . To determine whether amino-terminal truncation results in a redistribution of Dido3 in mitotic cells, we compared the subcellular localization of Dido3 and Dido3ΔNT by immunofluorescence (IF) with an antibody against the Dido3 carboxy terminus [28] , [30] . Whereas wild-type (WT) Dido3 has a predominantly nuclear localization, a large proportion of Dido3ΔNT localized to the cytosol in MEFs ( Fig. 1c ). Quantification of nuclear and cytosolic signals showed that approximately three times more Dido3ΔNT than WT Dido3 was present in the cytosol ( Fig. 1d ). These data indicate that the amino-terminal domains of Dido3 have a role in nuclear retention, and show an increased cytosolic availability of Dido3ΔNT compared with WT Dido3. To determine whether increased cytosolic level of Dido3ΔNT results in an increased accumulation at the basal body, we labelled WT and Dido3ΔNT MEF (hereafter ΔNT MEF) with antibodies against Ac-tub and Dido3 ( Fig. 1e,f ). Compared with WT cells, ΔNT MEF yielded a significantly higher signal at the cilium base ( Fig. 1g ), showing that redistribution of Dido3ΔNT to the cytosol increases the amount of protein at the basal body. Dido3 negatively control scilium size As the same organelle that sprouts the cilium in interphase organizes the mitotic spindle during cell division, cilia must be shortened and disassembled before mitosis [11] . The subcellular distribution and recruitment of Dido3 to spindle poles hint at a role for the protein in this process. To determine whether Dido3 has a role in the regulation of cilium size, we measured the primary cilium length in serum-starved WT and ΔNT MEF ( Fig. 2 ). Labelling with antibodies against the proliferation marker proliferating-cell nuclear antigen confirmed cell cycle arrest after serum starvation ( Supplementary Fig. 3 ). Although cell cycle arrest readily produced cilia in the WT and ΔNT MEFs ( Fig. 2a ), average cilium size was significantly reduced in the ΔNT MEF ( Fig. 2b ). As the independent marker ARL13B [34] distributed along, but did not extend significantly beyond the Ac-tub signal ( Fig. 2c,d ), Ac-tub accurately determined cilium size for WT and ΔNT MEF. Subsequent quantification revealed that cilium size negatively correlated with Dido3/Dido3ΔNT protein levels at the basal body ( Supplementary Fig. 4 ). As Dido3ΔNT is more efficiently recruited to the basal body than WT Dido3 ( Fig. 1 ), these data suggest that Dido3 negatively regulates cilium size. To confirm Dido3-dependent cilium size restriction in an alternative model, RNAi against Dido was expressed in retinal pigment epithelium (RPE) cells by lentiviral delivery ( Fig. 3 ). IF ( Fig. 3a ) and western blotting (WB) confirmed RNAi efficiency ( Fig. 3b ). Compared with RPE cells treated with mock interfering RNA, cells with reduced Dido levels had significantly larger cilia ( Fig. 3c ), and a small proportion of Dido RNAi cells carried extremely long cilia never found in mock-treated controls. ARL13B again confirmed that Ac-tub faithfully represented cilium size in Dido RNAi cells, even for extremely long cilia ( Fig. 3d,e ). Taken together, these results show that a Dido gene product exerts negative control over cilium length. 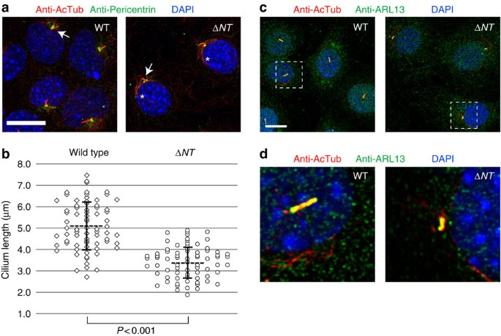Figure 2: Reduced cilium size in death inducer obliterator 3 (Dido3) ΔNT mouse embryonic fibroblasts (MEFs). (a) WT or ΔNT MEFs were seeded on coverslips, grown until confluent and serum starved. Subsequently, cells were labelled with anti-Pericentrin (green) and Ac-tub (red) antibodies, and counterstained for DNA (blue). Although WT and ΔNT MEFs formed cilia (arrows) at comparable frequencies, measurement of cilium length (b) showed significantly shorter cilia in ΔNT MEF (one-way analysis of variance). Horizontal dotted bar indicates average cilium size, error bars indicate standard error of the mean (n=72). Note the accumulation of acetylated microtubules adjacent to the nucleus in ΔNT MEFs (asterisk). (c) Immunofluorescence with anti-ARL13B antibodies (green) confirmed Ac-tub (red) as an accurate marker of cilium size. (d) Magnification of boxed areas inc. Scale bars, 10 μm. Separate grey scale versions of the micrograph images are supplied inSupplementary Fig. 13. Figure 2: Reduced cilium size in death inducer obliterator 3 (Dido3) ΔNT mouse embryonic fibroblasts (MEFs). ( a ) WT or ΔNT MEFs were seeded on coverslips, grown until confluent and serum starved. Subsequently, cells were labelled with anti-Pericentrin (green) and Ac-tub (red) antibodies, and counterstained for DNA (blue). Although WT and ΔNT MEFs formed cilia (arrows) at comparable frequencies, measurement of cilium length ( b ) showed significantly shorter cilia in ΔNT MEF (one-way analysis of variance). Horizontal dotted bar indicates average cilium size, error bars indicate standard error of the mean ( n =72). Note the accumulation of acetylated microtubules adjacent to the nucleus in ΔNT MEFs (asterisk). ( c ) Immunofluorescence with anti-ARL13B antibodies (green) confirmed Ac-tub (red) as an accurate marker of cilium size. ( d ) Magnification of boxed areas in c . Scale bars, 10 μm. Separate grey scale versions of the micrograph images are supplied in Supplementary Fig. 13 . 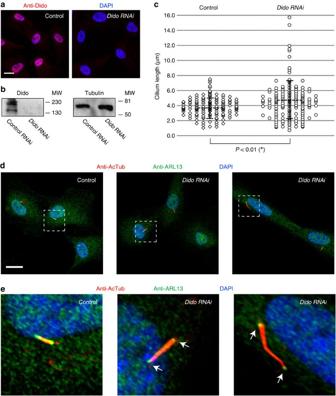Figure 3: Suppression ofDidoexpression increases cilium size. RPE-1 cells were transduced with lentiviral particles expressing a non-targeting RNA interference (RNAi) or an RNAi directed againstDido. Transduced cells were then seeded on glass coverslips, grown until confluent and serum starved. Immunofluorescence labelling (a) and western blotting (b) with antibodies against human death inducer obliterator (Dido) showed efficient suppression. Measurement of cilium length (c) showed thatDidosuppression resulted in significantly longer cilia (one-way analysis of variance). Horizontal dotted bar indicates average cilium size, error bars indicate standard error of the mean (n=58). Note: Outliers (cilia with length>8 μm) were excluded for calculation ofP-value. (d–g) Immunofluorescence with anti-ARL13B antibodies (green) confirmed Ac-tub (red) as an accurate marker of cilium size, even for extremely long cilia (right panel). (e) Magnification of boxed areas ind. Whereas ARL13B distributes evenly over the cilium in control cells, Dido RNAi causes redistribution to the cilium base and tip (arrows). Molecular weight of markers is indicated in kDa on the right of the western blots. Scale bars, 10 μm. Separate grey scale versions of the micrograph images are supplied inSupplementary Fig. 14. Full size image Figure 3: Suppression of Dido expression increases cilium size. RPE-1 cells were transduced with lentiviral particles expressing a non-targeting RNA interference (RNAi) or an RNAi directed against Dido . Transduced cells were then seeded on glass coverslips, grown until confluent and serum starved. Immunofluorescence labelling ( a ) and western blotting ( b ) with antibodies against human death inducer obliterator (Dido) showed efficient suppression. Measurement of cilium length ( c ) showed that Dido suppression resulted in significantly longer cilia (one-way analysis of variance). Horizontal dotted bar indicates average cilium size, error bars indicate standard error of the mean ( n =58). Note: Outliers (cilia with length>8 μm) were excluded for calculation of P -value. ( d – g ) Immunofluorescence with anti-ARL13B antibodies (green) confirmed Ac-tub (red) as an accurate marker of cilium size, even for extremely long cilia (right panel). ( e ) Magnification of boxed areas in d . Whereas ARL13B distributes evenly over the cilium in control cells, Dido RNAi causes redistribution to the cilium base and tip (arrows). Molecular weight of markers is indicated in kDa on the right of the western blots. Scale bars, 10 μm. Separate grey scale versions of the micrograph images are supplied in Supplementary Fig. 14 . Full size image The Dido gene codes for three isoforms, termed Dido1, -2 and -3. Of these, Dido3 is the most abundant and the only isoform that localizes to centrosomes [27] , [28] . The centrosomal localization and prevalence of Dido3 suggest that this isoform in particular might control the primary cilium. To analyse which Dido isoforms regulate cilium size, each V5-tagged isoform was overexpressed in RPE-1 cells ( Fig. 4 ). Whereas overexpression of Dido1 or Dido2 allowed for normal cilium formation and did not significantly change cilium size, overexpression of Dido3 significantly reduced cilium size ( Fig. 4a,b ). Regularly, Dido3 overexpression prevented cilium formation even though Ac-tub was detected in cytoplasmic microtubules ( Fig. 4c ). Quantification showed a significant reduction of cilium length in cells that overexpressed Dido3 ( Fig. 4d ). These results show that the Dido3 isoform in particular regulates cilium length, in agreement with its centrosomal targeting. 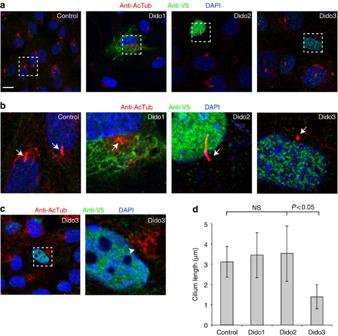Figure 4: Death inducer obliterator 3 (Dido3) overexpression reduces cilium size. RPE-1 cells were seeded on coverslips, transfected with plasmids expressing V5-tagged Dido1, -2 or -3, grown until confluence and serum starved. (a) Cells were labelled with antibodies against the V5-tag (green) and Ac-tub (red), and counterstained for DNA (blue). (b) Magnification of boxed areas ina. Regularly, Dido3 overexpression prevented cilium formation altogether (c), even though perinuclear microtubules are acetylated (arrowhead). Measurement of cilium length (d) showed that overexpression of Dido3, but not that of Dido1 or -2, significantly reduced cilium size (one-way analysis of variance). Error bars indicate standard error of the mean (n=8). Scale bar, 10 μm. Separate grey scale versions of the micrograph images are supplied inSupplementary Fig. 15. Figure 4: Death inducer obliterator 3 (Dido3) overexpression reduces cilium size. RPE-1 cells were seeded on coverslips, transfected with plasmids expressing V5-tagged Dido1, -2 or -3, grown until confluence and serum starved. ( a ) Cells were labelled with antibodies against the V5-tag (green) and Ac-tub (red), and counterstained for DNA (blue). ( b ) Magnification of boxed areas in a . Regularly, Dido3 overexpression prevented cilium formation altogether ( c ), even though perinuclear microtubules are acetylated (arrowhead). Measurement of cilium length ( d ) showed that overexpression of Dido3, but not that of Dido1 or -2, significantly reduced cilium size (one-way analysis of variance). Error bars indicate standard error of the mean ( n =8). Scale bar, 10 μm. Separate grey scale versions of the micrograph images are supplied in Supplementary Fig. 15 . Full size image Dido3 controls intracellular HDAC6 distribution Tubulin deacetylation by HDAC6 has a major role in coordinating disassembly of the primary cilium with the cell cycle [11] . HDAC6 has unique substrate specificity for nonhistone proteins [35] and associates with a variety of nuclear and cytoplasmic structures, including transcription factor complexes [36] , microtubules [18] and the actin cytoskeleton [23] . Nonetheless, few details about the mechanisms that govern targeting of HDAC6 to its various sites of action are known. To study a possible role of Dido3 in HDAC6 localization, we compared the subcellular distribution of HDAC6 in proliferating WT and ΔNT MEF ( Fig. 5 ). In WT MEF, where Dido3 has a mostly nuclear localization, HDAC6 distributed over the nucleus and cytoplasm. The ΔNT MEF, however, in which Dido3ΔNT has a more cytosolic distribution, indicated a more cytoplasmic HDAC6 pattern, especially pronounced at the perinuclear region and cell periphery ( Fig. 5a ). Subcellular fractionation and blotting with anti-HDAC6 antibodies confirmed an increase of cytosolic deacetylase levels in ΔNT MEF ( Fig. 5b ). These data indicate that the relocalization of Dido3ΔNT with respect to Dido3 results in HDAC6 redistribution to the cytoplasm, and suggests that Dido3 has a role in HDAC6 targeting. Protein co-precipitation experiments using glutathione S -transferase (GST)-tagged Dido corroborated a role for Dido3 in HDAC6 targeting ( Fig. 5b ). Mass spectrometry identified α-tubulin, β-tubulin and actin in protein complexes that co-purified with GST-Dido ( Supplementary Fig. 5 ), and WB identified associated HDAC6 ( Fig. 5c ). Coexpression and immunoprecipitation with antibodies against HA-tagged HDAC6 co-precipitated a small but reproducible amount of V5-tagged Dido3 ( Supplementary Fig. 6 ). The identified proteins bound to the central domains of Dido3; whereas the amino-terminal domain governs histone interaction [30] , and the carboxy terminus targets the protein to the centrosome ( Supplementary Fig. 1 ), the central region participates in the actual cargo binding. Taken together, these results show a role for Dido3 in the subcellular targeting of HDAC6. 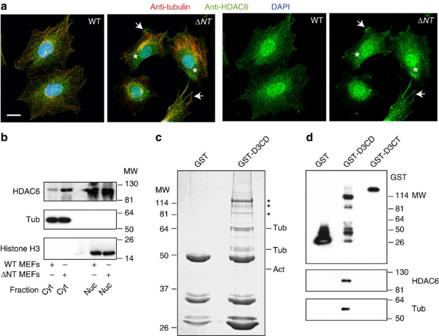Figure 5: Death inducer obliterator 3 (Dido3) controls histone deacetylase 6 (HDAC6) distribution. (a) Wild-type (WT) or ΔNT mouse embryonic fibroblasts (MEFs) were seeded on coverslips, labelled with antibodies against HDAC6 (green) and tubulin (red), and counter stained DNA (blue). HDAC6 distributes over the nucleus and cytoplasm in WT and ΔNT MEFs, but ΔNT MEF show increased levels of HDAC6 in the perinuclear region (asterisks) and cell periphery (arrows). Scale bar, 10 μm. (b) Cytosolic and nuclear fractions isolated from WT or ΔNT MEFs were separated by SDS–polyacrylamide gel electrophoresis (SDS–PAGE), and identified with antibodies against tubulin and histone H3, respectively. Western blotting with anti-HDAC6 antibodies revealed increased HDAC6 levels in the cytosolic fraction of ΔNT MEF as compared with WT MEF. (c) Pull-down experiments using glutathioneS-transferase (GST) fused to the central domains of Dido3 (GST-D3CD,Supplementary Fig. 2). GST and GST-D3CD were purified from HEK293T cells and analysed by SDS–PAGE and Coomassie staining. Proteomics analysis of isolated bands identified tubulin (Tub) and actin (Act) as principal interacting proteins. Asterisks indicate partial proteolysis of the GST fusion and association with endogenous Dido1 (ref.26). (d) Western blotting with anti-GST, anti-tubulin and anti-HDAC6 antibodies showed co-purification of HDAC6 and the central domains of Dido3. No binding to GST or the centrosomal targeting domain (GST-D3CT,Supplementary Fig. 2) was detected. Molecular weight of markers is indicated in kDa on the left (c) or right (b,d). Figure 5: Death inducer obliterator 3 (Dido3) controls histone deacetylase 6 (HDAC6) distribution. ( a ) Wild-type (WT) or ΔNT mouse embryonic fibroblasts (MEFs) were seeded on coverslips, labelled with antibodies against HDAC6 (green) and tubulin (red), and counter stained DNA (blue). HDAC6 distributes over the nucleus and cytoplasm in WT and ΔNT MEFs, but ΔNT MEF show increased levels of HDAC6 in the perinuclear region (asterisks) and cell periphery (arrows). Scale bar, 10 μm. ( b ) Cytosolic and nuclear fractions isolated from WT or ΔNT MEFs were separated by SDS–polyacrylamide gel electrophoresis (SDS–PAGE), and identified with antibodies against tubulin and histone H3, respectively. Western blotting with anti-HDAC6 antibodies revealed increased HDAC6 levels in the cytosolic fraction of ΔNT MEF as compared with WT MEF. ( c ) Pull-down experiments using glutathione S -transferase (GST) fused to the central domains of Dido3 (GST-D3CD, Supplementary Fig. 2 ). GST and GST-D3CD were purified from HEK293T cells and analysed by SDS–PAGE and Coomassie staining. Proteomics analysis of isolated bands identified tubulin (Tub) and actin (Act) as principal interacting proteins. Asterisks indicate partial proteolysis of the GST fusion and association with endogenous Dido1 (ref. 26 ). ( d ) Western blotting with anti-GST, anti-tubulin and anti-HDAC6 antibodies showed co-purification of HDAC6 and the central domains of Dido3. No binding to GST or the centrosomal targeting domain (GST-D3CT, Supplementary Fig. 2 ) was detected. Molecular weight of markers is indicated in kDa on the left ( c ) or right ( b , d ). Full size image Dido3 modulates HDAC6 targeting and tubulin acetylation As Ac-tub is an important HDAC6 substrate [18] , [19] , Dido3-dependent HDAC6 redistribution might direct the deacetylation of this cytoplasmic protein. Detection of Ac-tub indeed revealed reduced tubulin acetylation in ΔNT MEF, where Dido and HDAC6 redistributed to the cytoplasm ( Fig. 6a ). In contrast to ΔNT MEF, which have increased cytoplasmic Dido3 levels, a reduction of Dido expression by RNAi increased tubulin acetylation ( Fig. 6b ). As the acetylated lysine recognized by the anti-Ac-tub antibody is located on the inside of microtubules [37] , tubulin polymerization is thought to shield this residue from HDAC6. Correspondingly, Nocodazole treatment—a compound that disassembles microtubules—reduced tubulin acetylation, whereas Taxol treatment—which polymerizes and bundles tubulin—increased Ac-tub levels, thereby minimizing the differences between WT and ΔNT MEF ( Fig. 6a ). In addition to the primary cilium, which harbors almost all Ac-tub in WT MEF, acetylated microtubules were frequently found adjacent to the nucleus in ΔNT MEF ( Fig. 2 , Supplementary Fig. 7A ). These data suggest that ΔNT MEF respond to increased HDAC6 activity by increasing tubulin acetylation, excluding reduced acetylation as a cause of lower Ac-tub levels. Small-molecule inhibition of HDAC6 (ref. 38 ) increased Ac-tub levels in WT and ΔNT MEF ( Fig. 6c , Supplementary Fig. 7B ), confirming the role of HDAC6. Under these conditions, Ac-tub levels rose considerably higher in ΔNT MEF than in WT MEF, corroborating the hypothesis that increased tubulin acetylation partially compensates for HDAC6 redistribution. 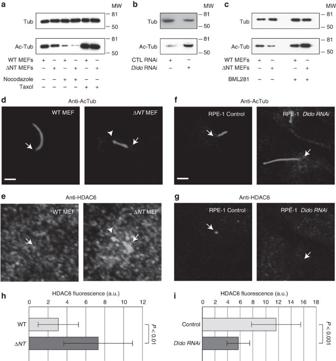Figure 6: Death inducer obliterator 3 (Dido3) directs histone deacetylase 6 (HDAC6) to cilia and modulates tubulin acetylation. (a) WT or ΔNT mouse embryonic fibroblasts (MEFs) were treated for 60 min with Nocodazole or Taxol as indicated. Cells were then lysed and analysed by western blotting with antibodies against tubulin or Ac-tub. Compared with WT cells, ΔNT MEF showed reduced levels of tubulin acetylation in untreated controls or when microtubules were depolymerized. Forced polymerization of microtubules overcame increased tubulin deacetylation. (b) Retinal pigment epithelium (RPE)-1 cells treated with RNA interference (RNAi) againstDidoshowed increased tubulin acetylation compared with mock-transduced cells. (c) The HDAC6 inhibitor BML-281 overcomes increased tubulin deacetylation in ΔNT MEFs; whereas dimethylsulphoxide (DMSO) vehicle-treated ΔNT MEF showed low Ac-tub levels compared with WT controls, BML-281 reversed this effect, suggesting compensation by additional tubulin acetylation. (d) Redistribution of Dido3 in ΔNT MEF causes accumulation of centrosomal HDAC6. WT or ΔNT MEFs were treated as inFig. 2, and labelled for Ac-tub (d) and HDAC6 (e). Centrosomal regions at the cilium base are indicated with an arrow, and HDAC6 accumulation at the cilium tip with an arrowhead. (f) RNAi suppression ofDidoresults in HDAC6 loss from the centrosome. RPE-1 cells were treated as inFig. 3a, and labelled for Ac-tub (g) and HDAC6 (f). Corresponding colour overviews are available in theSupplementary Information. (h,i) Quantification of HDAC6 levels at the cilium base indandf, respectively, by one-way analysis of variance. Error bars indicate standard error of the mean (h,n=15;i,n=40). Molecular weight of markers is indicated in kDa on the right of the western blots. Scale bars, 2 μm. Figure 6: Death inducer obliterator 3 (Dido3) directs histone deacetylase 6 (HDAC6) to cilia and modulates tubulin acetylation. ( a ) WT or ΔNT mouse embryonic fibroblasts (MEFs) were treated for 60 min with Nocodazole or Taxol as indicated. Cells were then lysed and analysed by western blotting with antibodies against tubulin or Ac-tub. Compared with WT cells, ΔNT MEF showed reduced levels of tubulin acetylation in untreated controls or when microtubules were depolymerized. Forced polymerization of microtubules overcame increased tubulin deacetylation. ( b ) Retinal pigment epithelium (RPE)-1 cells treated with RNA interference (RNAi) against Dido showed increased tubulin acetylation compared with mock-transduced cells. ( c ) The HDAC6 inhibitor BML-281 overcomes increased tubulin deacetylation in ΔNT MEFs; whereas dimethylsulphoxide (DMSO) vehicle-treated ΔNT MEF showed low Ac-tub levels compared with WT controls, BML-281 reversed this effect, suggesting compensation by additional tubulin acetylation. ( d ) Redistribution of Dido3 in ΔNT MEF causes accumulation of centrosomal HDAC6. WT or ΔNT MEFs were treated as in Fig. 2 , and labelled for Ac-tub ( d ) and HDAC6 ( e ). Centrosomal regions at the cilium base are indicated with an arrow, and HDAC6 accumulation at the cilium tip with an arrowhead. ( f ) RNAi suppression of Dido results in HDAC6 loss from the centrosome. RPE-1 cells were treated as in Fig. 3a , and labelled for Ac-tub ( g ) and HDAC6 ( f ). Corresponding colour overviews are available in the Supplementary Information . ( h , i ) Quantification of HDAC6 levels at the cilium base in d and f , respectively, by one-way analysis of variance. Error bars indicate standard error of the mean ( h , n =15; i , n =40). Molecular weight of markers is indicated in kDa on the right of the western blots. Scale bars, 2 μm. Full size image HDAC6 has an important role in the deacetylation of ciliary Ac-tub at the time of cilium disassembly in mitotic cells [11] . As Dido3 negatively regulates cilium size, localizes to the basal body and modulates HDAC6 distribution, it might also control HDAC6 at the primary cilium. To further evaluate the role of Dido3 in protein targeting, HDAC6 levels at the basal body were examined in growth-arrested cells ( Fig. 6d–g , Supplementary Fig. 8 ). Whereas HDAC6 levels were comparable to that of the surrounding cytoplasm in WT MEFs, the deacetylase was more abundant around the cilium base in ΔNT MEFs ( Fig. 6d,e ), suggesting that Dido3-dependent targeting controls ciliary HDAC6 levels. The working model of mitotic cilium resorption comprises transport of HDAC6 along the ciliary microtubules [11] . In agreement with this model and with Dido3-dependent targeting of HDAC6 to the cilium base, the apical tips of cilia in ΔNT MEFs commonly showed marked amounts of the deacetylase ( Fig. 6e , arrowhead). RNAi in RPE-1 cells confirmed the role of Dido in protein targeting; whereas HDAC6 consistently accumulated at the basal body in control cells, the protein was lacking from this organelle in cells with reduced Dido expression ( Fig. 6f,g ). Quantification revealed significant changes in the amount of HDAC6 at the basal body ( Fig. 6h,i ), which followed the observed changes in Dido3 levels, and double labelling with antibodies against Ac-tub showed an inverse correlation between the amount of deacetylase at the basal body and cilium size ( Supplementary Fig. 9 ). Taken together, these results show that Dido3-dependent HDAC6 targeting negatively regulates cilium size in growth-arrested cells. The actin network maintains localization of Dido3 and HDAC6 In addition to HDAC6 levels, filamentous actin has a limiting effect on cilium formation [15] . Whereas HDAC6 initially has been associated with mitotic cilium disassembly [11] , actin polymerization controls cilium size in cell cycle-arrested cells. As the GST-D3CD fusion bound actin in addition to tubulin, the actin cytoskeleton might regulate the effect of Dido3 and HDAC6 on cilia. Double labelling with Phalloidin and antibodies against Dido3 or HDAC6 confirmed recruitment of the two proteins to the actin cytoskeleton, which was more pronounced in ΔNT MEFs compared with WT MEFs ( Supplementary Figs 10 and 11 ). To study a possible relation between actin polymerization and tubulin acetylation, integrity of the actin network in WT and ΔNT MEFs was disrupted with cytochalasin D [15] . Whereas cytochalasin D treatment had little effect on tubulin acetylation in WT MEFs, it partially restored Ac-tub levels in ΔNT MEFs ( Fig. 7a ). Although cytochalasin D increased cilium size in WT and ΔNT MEF, it had a greater effect on ΔNT MEFs ( Fig. 7b ); cilium size in mock-treated ΔNT MEF was significantly smaller than that of WT MEF, but cilium size in cytochalasin D-treated WT and ΔNT MEFs did not differ significantly. These results indicate that actin depolymerization overcomes increased HDAC6 targeting to the basal body. As a proportion of Dido3 and HDAC6 is associated with the actin cytoskeleton ( Supplementary Figs 10 and 11 ), the actin network might maintain localization of these proteins at the basal body. To analyse the role of the actin network in Dido3 and HDAC6 targeting, these proteins were detected by IF after cytochalasin D treatment ( Fig. 7c–f ). Disruption of the actin network resulted in the loss of Dido3 ( Fig. 7c,d ) and HDAC6 ( Fig. 7e,f ) from the basal body, concomitant with cilium elongation. These results indicate a role for the actin network in Dido3 and HDAC6 targeting, and suggest a link between cilium size regulation in mitotic and in growth-arrested cells. 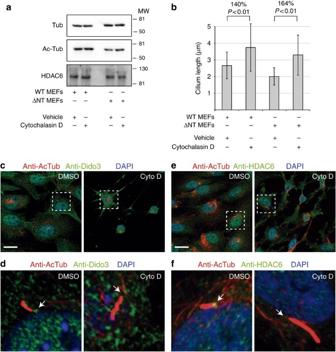Figure 7: The actin cytoskeleton maintains localization of death inducer obliterator 3 (Dido3) and histone deacetylase 6 (HDAC6). WT or ΔNT mouse embryonic fibroblasts (MEFs) were treated with cytochalasin D or dimethylsulphoxide (DMSO) vehicle for 2 h. Cells were then lysed and analysed by western blotting with antibodies against tubulin, Ac-tub and HDAC6. (a) Whereas cytochalasin D treatment had little effect on WT MEF, it caused a partial recovery of tubulin acetylation in ΔNT MEF. Thus, actin depolymerization partially overcomes increased tubulin deacetylation in these cells. Molecular weight markers are indicated in kDa on the right. (b) WT or ΔNT MEFs were grown as inFig. 2a, and treated as ina. Cells were then labelled with antibodies against Ac-tub. Quantification of cilium length (one-way analysis of variance) revealed a significant cilium elongation after actin depolymerization, which was more pronounced in ΔNT MEF than in WT MEF. Error bars indicate standard error of the mean (n=60). Cytochalasin D treatment resulted in loss of Dido3 (c,d) and HDAC6 (e,f) from the centrosome, suggesting that the actin network controls cilium length by protein targeting to the basal body.(d,f) Magnification of boxed areas incande, respectively. Scale bars, 10 μm. Separate grey scale versions of the micrograph images are supplied inSupplementary Fig. 16. Figure 7: The actin cytoskeleton maintains localization of death inducer obliterator 3 (Dido3) and histone deacetylase 6 (HDAC6). WT or ΔNT mouse embryonic fibroblasts (MEFs) were treated with cytochalasin D or dimethylsulphoxide (DMSO) vehicle for 2 h. Cells were then lysed and analysed by western blotting with antibodies against tubulin, Ac-tub and HDAC6. ( a ) Whereas cytochalasin D treatment had little effect on WT MEF, it caused a partial recovery of tubulin acetylation in ΔNT MEF. Thus, actin depolymerization partially overcomes increased tubulin deacetylation in these cells. Molecular weight markers are indicated in kDa on the right. ( b ) WT or ΔNT MEFs were grown as in Fig. 2a , and treated as in a . Cells were then labelled with antibodies against Ac-tub. Quantification of cilium length (one-way analysis of variance) revealed a significant cilium elongation after actin depolymerization, which was more pronounced in ΔNT MEF than in WT MEF. Error bars indicate standard error of the mean ( n =60). Cytochalasin D treatment resulted in loss of Dido3 ( c , d ) and HDAC6 ( e , f ) from the centrosome, suggesting that the actin network controls cilium length by protein targeting to the basal body. ( d , f ) Magnification of boxed areas in c and e , respectively. Scale bars, 10 μm. Separate grey scale versions of the micrograph images are supplied in Supplementary Fig. 16 . Full size image The proper control of cilium formation, maintenance and disassembly are thought critical for a wide range of cellular processes, but we are just starting to uncover the mechanisms that govern control of this organelle. The variety of processes in which the cilium intervenes is reflected by the complexity of its regulation, which involves cell cycle regulators, extracellular signals, centriole migration and actin remodelling, among others [3] . One of the most striking features of the primary cilium is its capacity to respond to the cell cycle [11] as well as adapt its size to the needs of non-proliferating cells [15] , [17] . Nonetheless, if and how different control mechanisms converge on cilium size remain largely unknown. Here, we show that Dido3 controls cilium size by regulating availability of HDAC6 at the centrosome. Compared with other deacetylases, HDAC6 participates in a broad range of cellular activities and for this reason is enriched in the corresponding subcellular locations [11] , [23] , [25] , [39] . This uneven subcellular distribution suggests control mechanisms in addition to the kinase-dependent activation that was described before [11] , [25] , but no proteins involved in HDAC6 targeting have been identified so far. Interference with Dido3 distribution or levels leads to alterations of HDAC6 in the cytoplasm and subsequent changes in tubulin acetylation in growth-arrested cells. This effect on tubulin acetylation additionally depends on the actin cytoskeleton, which itself has been shown to control steady-state cilium size [15] . In agreement with the role of the actin cytoskeleton, actin depolymerization resulted in a loss of Dido3 and HDAC6 localization in our experiments. In contrast to the switch-like kinase cascade that controls HDAC6 activation in mitosis [11] , local concentration changes of the deacetylase provide cells with a gradual regulation of cilium length ( Fig. 8 ). The small but reproducible amount of co-precipitated protein in the immunoprecipitations is compatible with a transient interaction model, in which Dido3 promotes HDAC6 delivery to the cilium base but is dispensable for further transport along the stalk. RNAi depletion of Dido3 caused a reduction of HDAC6 at the basal body and a concomitant lengthening of cilia. Only in a small proportion of cells, however, cilium size reached a multiple of the normal length. Given the nature of RNAi, incomplete Dido3 depletion might result in partial lengthening because of residual HDAC6 delivery. Surprisingly, cilia of extreme length showed uneven ARL13B distribution ( Fig. 3d,e ). Possibly, tubulin hyperacetylation affects intraciliary transport, causing depletion of ARL13B along the stalk and accumulation at the base and tip. 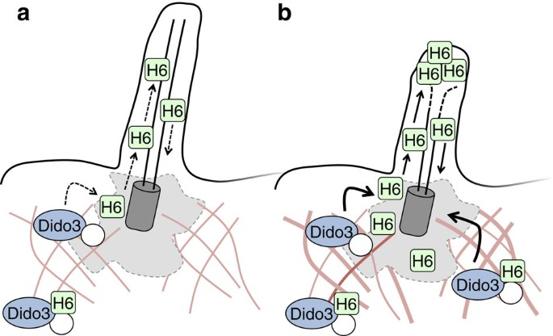Figure 8: Working model of death inducer obliterator 3 (Dido3)-dependent histone deacetylase 6 (HDAC6) targeting. (a) Basal levels of Dido3 (blue) and HDAC6 (green) maintain a steady state in which cilium growth and resorption are in equilibrium. (b) Increased recruitment of Dido3 to the basal body, for example, through the buildup of actin fibres (red) or liberation from the nucleus, results in higher local concentrations of HDAC6. Subsequent intraciliary transport directs HDAC6 to the apical tip, where tubulin deacetylation promotes a gradual reduction of cilium size. Figure 8: Working model of death inducer obliterator 3 (Dido3)-dependent histone deacetylase 6 (HDAC6) targeting. ( a ) Basal levels of Dido3 (blue) and HDAC6 (green) maintain a steady state in which cilium growth and resorption are in equilibrium. ( b ) Increased recruitment of Dido3 to the basal body, for example, through the buildup of actin fibres (red) or liberation from the nucleus, results in higher local concentrations of HDAC6. Subsequent intraciliary transport directs HDAC6 to the apical tip, where tubulin deacetylation promotes a gradual reduction of cilium size. Full size image Although our results indicate a role of Dido3 in cilium control, this does not exclude involvement of other regulatory proteins or mechanisms—small-molecule inhibition hints at acetyltransferases, and the Dido1 and Dido2 isoforms might reduce Dido3 anchoring to the chromatin [31] —in cilium length regulation. One of the additional mechanisms to control cilium size, identified recently, is autophagy [40] , [41] . As both cilium elongation and shortening have been attributed to autophagy, the exact relation between the two remains to be determined. Interestingly, however, HDAC6 has a central role in autophagy too [22] , [42] , suggesting a coordinating role for protein deacetylation. Future identification of the key substrates of HDAC6 in ciliogenesis and autophagy might help to elucidate connections between these two processes. Our results indicate that HDAC6 is regulated by a combination of subcellular distribution in addition to spatiotemporal activation; a subpopulation of HDAC6 is phosphorylated by kinases that accumulate at the basal body in a cell cycle-dependent manner [11] , [25] . Steady state and mitotic control of the cilium thus converge at the level of HDAC6. Dido3 itself might function in a way that is comparable to HDAC6; whereas Dido3 mostly localizes to the nucleus in interphase, the protein accumulates at the spindle poles in cell division [28] . Dido3 distribution is determined in part by its binding to trimethylated lysine 4 in histone H3, and a truncation mutant has reduced histone binding in vivo [30] . Consequently, our results showed higher availability of Dido3 and HDAC6 at the centrosome in this mutant. Remarkably, histone H3 residues adjacent to lysine 4 are phosphorylated when chromosomes condense in early mitosis [43] ; this phosphorylation leads to redistribution of Dido3 from the chromatin to centrosomes [31] . As histone H3 phosphorylation depends on the same family of kinases that regulate cilium resorption, mitotic Dido3 redistribution might prime the cilium with HDAC6 for subsequent kinase activation. Taken together, our results suggest that a highly integrated regulatory network controls the primary cilium and mitotic spindle. Cell culture WT and ΔNT MEFs [28] , and 3T3 cells were cultured in DMEM supplemented with 10% fetal calf serum and antibiotics. RPE-1 cells (ATCC CRL-4000) were cultured in DMEM+F12 (1:1) supplemented with 10% fetal calf serum and antibiotics. Dido RNAi knockdown For the knockdown of protein expression, small hairpin RNA against human (sc-35194-v) or mouse (sc-35195-v) Dido was delivered by lentiviral particles (Santa Cruz Biotechnology). A scrambled non-targeting RNA (sc-108080) was used as control. 2 × 10 5 cells were transduced with 2 × 10 5 particles (multiplicity of infection=1), following the manufacturers’ instructions. One day after viral transduction, cells were selected with 5 μg ml −1 puromycin for 72 h, and then plated on glass coverslips for further experiments. Reagents and transfections Antibodies against mouse Dido3 have been described before [28] , [30] , and were used in a 1:150 dilution. Antibodies against GST (sc-138, 1:1,000 dilution for WB) were from Santa Cruz Biotechnology, antibodies against α/β-tubulin (DM1a/DM1b,1:1,000 dilution for WB, 1:500 dilution for IF) and Ac-tub (6-11B-1, 1:1,000 dilution for WB, 1:500 dilution for IF) were from Sigma, and antibodies against human Dido (ab92868, 1:500 dilution for WB, 1:200 dilution for IF), HDAC6 (ab1440, 1:1,000 dilution for WB, 1:200 dilution for IF) [44] , [45] , Pericentrin (ab4448, 1:200 dilution for IF), ARL13B (ab83879, 1:200 dilution for IF), histone H3 (ab1791, 1:1,000 dilution for WB), the HA tag (ab9110, 1:1,000 dilution for WB) and the V5 tag (ab9116, 1:1,000 dilution for WB, 1:200 dilution for IF) were from Abcam. The HDAC6 inhibitor BML-281 (ref. 38 ) was from Enzo Life Sciences (Farmingdale, NY, USA) and applied in a final concentration of 0.1 μM for 16 h. Cytochalasin D (Sigma) was used at a final concentration of 0.5 μM for 30 min as described elsewhere [16] . For fractionation, MEFs (10 6 cells) were grown to confluence, and subcellular fractions were isolated with a nuclear-cytosol fractionation kit (JM-K266, MBL) according to the manufacturer’s instructions. Additional uncropped images of WBs and colour separations of IF are available in Supplementary Figs 19–21 . To generate plasmids encoding V5-tagged Dido proteins, a custom synthetic DNA comprising a Kozak sequence and triple V5 peptides (Life Technologies) was fused to the amino-terminus of mouse Dido1 (ref. 26 ), Dido2 or Dido3 cDNA [27] and expressed from pcDNA3 (Life Technologies). For transient transfections, 2 × 10 5 RPE-1 or 3T3 cells were seeded on glass coverslips in a six-well tissue culture plate. After 24 h, transfections were performed using 6 μl XtremeGENE 9 (Roche) and 2 μg of plasmid DNA, as recommended by the manufacturer. Cells were analysed by IF 24 h after transfection for subcellular localization, or after an additional 48 h serum starvation [9] for measurement of cilium size. GST pull-downs and protein identification To construct the GST fusions, Dido3 (ref. 27 ) cDNA fragments flanked by Bgl II and Xho I sites were cloned into the same sites of pEBG [46] . A fragment corresponding to amino acids 530–1175 was used for the Dido3 central domain, and a fragment corresponding to amino acids 1176–2256 for the carboxy-terminal domain. GST fusions were purified essentially as described [47] . Briefly, fusion constructs were transfected into HEK293T cells, and expression was allowed for 48 h. Cells were collected, resuspended in binding buffer (20 mM Tris-HCl pH 7.9, 180 mM KCl, 1 mM dithiothreitol, 1 mM Pefabloc SC (Roche), 0.05% NP-40 and 0.1% BSA) and lysed by sonication. After clearing debris (10,000 × g , 10 min, 4 °C), 750 μg of cell lysate were incubated (2 h, 4 °C) with glutathione Sepharose (Amersham Pharmacia). After binding, columns were washed six times with wash buffer (binding buffer without BSA) and eluted with sample buffer. Proteins were separated by 12% SDS–PAGE and detected by WB or Coomassie Brilliant Blue staining. For protein identification from Coomassie-stained gels, all bands detected were excised and washed with distilled water. After overnight trypsin digestion, samples were purified and concentrated on a C18 Zip Tip (Millipore). Peptides were eluted with 1.5 μl of a saturated solution of α-cyano-4-hydroxycinnamic acid in 50% acetonitrile/water (v/v) containing 0.1% trifluoroacetic acid (TFA) and analysed by matrix-assisted laser desorption-ionization time-of-flight mass spectrometry on an ABI4800 analyzer (Life Technologies). At least 100 scans were summed to obtain each spectrum. Database searches were performed using MASCOT at Matrix Science (http:// www.matrixscience.com ). IF and cilium length measurement Primary cilia were induced by serum starvation-induced growth arrest as described elsewhere [11] , [32] . Briefly, cells were grown on glass coverslips until 70% confluent, and growth medium was replaced by serum-free medium for 48–72 h. For IF, cells were rinsed in PBS, fixed in PBS containing 4% formaldehyde, and permeabilized in PBS with 0.5% Triton X-100. After blocking in PBS containing 1% bovine serum albumin (1 h, room temperature), cells were incubated with primary antibodies (1 h, room temperature). Cells were then washed, incubated with secondary antibodies (Jackson Immunoresearch), washed again and mounted in Prolong Gold antifade (Invitrogen). Confocal microscopy was performed using on an IX81 microscope (Olympus, Tokyo, Japan) with sequential excitation of fluorophores. ImageJ software ( http://rsbweb.nih.gov/ij/ ) was used for image processing and measurements. Representative images are shown in all figures. Cilium length was determined by Ac-tub labelling, followed by maximum projection and direct measurement, and levels of basal body-associated proteins were determined in 3 × 3 μm 2 surrounding the cilium base after adding upconfocal planes. Statistical analysis (duplicate experiments) by one-way analysis of variance was performed using SPSS Win 12.0 software (SPSS). How to cite this article: de Diego, A. S. et al. Dido3-dependent HDAC6 targeting controls cilium size. Nat. Commun. 5:3500 doi: 10.1038/ncomms4500 (2014).